Protrusion force microscopy reveals oscillatory force generation and mechanosensing activity of human macrophage podosomes Podosomes are adhesion structures formed in monocyte-derived cells. They are F-actin-rich columns perpendicular to the substrate surrounded by a ring of integrins. Here, to measure podosome protrusive forces, we designed an innovative experimental setup named protrusion force microscopy (PFM), which consists in measuring by atomic force microscopy the deformation induced by living cells onto a compliant Formvar sheet. By quantifying the heights of protrusions made by podosomes onto Formvar sheets, we estimate that a single podosome generates a protrusion force that increases with the stiffness of the substratum, which is a hallmark of mechanosensing activity. We show that the protrusive force generated at podosomes oscillates with a constant period and requires combined actomyosin contraction and actin polymerization. Finally, we elaborate a model to explain the mechanical and oscillatory activities of podosomes. Thus, PFM shows that podosomes are mechanosensing cell structures exerting a protrusive force. Macrophages play important roles in cellular immunity as well as tissue homeostasis during development and tissue repair. They can migrate through tissues with a large diversity of extracellular matrices that differ in several aspects including architecture, composition and elasticity. Cellular mechanosensing consists in probing the environment and influences cell decisions regarding functions such as migration, differentiation and morphogenesis. Numerous studies have focused on understanding how focal adhesions (FAs) exert traction forces onto the substratum using a variety of techniques known as traction force microscopy, where markers of substrate deformation (such as embedded microbeads, microprinted patterns or flexible micropillars…) [1] are tracked and their displacements converted into forces. Podosomes are another adhesion structures suspected to play a role in mechanosensing, as podosome-related structures, invadopodia from breast cancer cells and podosome rosettes formed in genetically modified fibroblasts have been shown to sense the environment stiffness [2] , [3] , [4] , [5] , [6] , [7] . Podosomes are present in monocytic lineage derivatives such as macrophages, dendritic cells and osteoclasts and are involved in cell migration and matrix degradation. Podosomes are F-actin-rich cone-shaped structures of ~600 nm height and submicron diameter, located at the basal face of cells, perpendicular to, and in contact with the substratum via integrins at the podosome ring [8] , [9] . Recently, super-resolution imaging of the adhesion ring revealed that its components are organized in clusters forming a polygonal structure [10] , [11] , [12] . Podosomes are regularly spaced and interconnected through a radial F-actin network [13] , [14] . They are very dynamic with a typical lifespan of 10 min, they display an actin turnover of ~30 s and periodical oscillations of core stiffness that depend on F-actin dynamics and myosin II activity [8] , [15] , [16] . To sense the environment, podosomes are predicted to exert perpendicular forces to the substratum by forming protrusions into the underlying matrix [17] , [18] , [19] . Although previous works from our lab and others have already shown that podosomes are oscillatory cell structures and have proposed that protrusion forces are applied at podosomes, none of these papers have been able to show podosomes dynamically protruding into a substrate and to measure the protrusion forces [8] , [18] . To the best of our knowledge, no method has been designed to evaluate protrusion forces exerted by a cell structure on a substratum. Here we develop an original approach that we call protrusion force microscopy (PFM) by analogy with traction force microscopy. This method involves the use of atomic force microscopy (AFM) that allows high spatial resolution and a temporal resolution compatible with cytoskeleton dynamics. PFM consists in measuring local protrusions generated onto a compliant Formvar sheet by macrophage podosomes. The protrusive forces generated by a podosome were then estimated using a model accounting for the mechanical properties of the Formvar membrane, and we showed that this oscillating protrusive force is controlled by cytoskeleton-related molecular motors. Finally, a model was designed to integrate F-actin dynamics and myosin II activity in the protruding activity of podosomes and its dynamics. PFM allows dynamic protrusion force measurement To quantify podosome protrusions into the substratum [17] , [18] , [19] , we designed an original method that we named PFM. It consists in measuring dynamic nanoscale strains caused by living human macrophages derived from blood monocytes on a compliant Formvar sheet using AFM. Formvar membranes were placed on a 90-μm-wide square mesh grid and mounted upside down after macrophage plating ( Fig. 1a ; Supplementary Fig. 1a,b ). AFM analysis of the opposite surface of the Formvar sheets revealed bulges (from ~10 to 50 nm high; Fig. 1b,d ) that formed beneath podosomes as shown by correlative AFM and fluorescence microscopy of podosome markers ( Fig. 1c ). On this substrate, macrophages formed podosomes with an organization and stiffness identical to podosomes developed by macrophages plated on glass ( Fig. 1c ; Supplementary Fig. 1c ). In addition, we verified that the bulges facing podosomes were not generated by experimental biases due to the AFM tip, that is, the topography of macrophage nanoscale footprints was not modified by varying the force exerted by the AFM cantilever tip onto the Formvar sheet ( Supplementary Fig. 1d ). Thus, we could conclude that the bulges observed on the Formvar sheet landscape were protrusions of the substratum generated by an actual protrusive activity of podosomes themselves. The mean height of protrusions measured for hundreds of podosomes was equal to 16.5±9.5 nm ( Fig. 1d ). Then, we reasoned that we could estimate the value of the protrusive force ( F ) generated by a single podosome by fitting the shape of a protrusion ( Fig. 1e ) with a mechanical model of the podosome. For this purpose, we first measured the biaxial Young’s modulus E /(1− υ 2 ) and residual tensile stress σ 0 of the Formvar sheet with an AFM, using a point-deflection method and deformations both higher and lower than podosome-induced protrusions ( Supplementary Note 1 ; Supplementary Fig. 2a,b ). Then, using a model of a circular clamped membrane under a punctual force in its centre, we determined the theoretical profile of the expected deformation and showed that this simplified model gives a good estimation of the actual podosome core protruding force. These mechanical studies led to a simplified and unified equation to calculate the force F from the radius ( a ) and the height ( h max ) of the protrusion only (see Fig. 1e ; Supplementary Note 2 ; Supplementary equation (7) ). The mean of the resulting values of F was equal to 94±59 nN ( Fig. 1f ). With this model, the radius of the circular membrane deformed by a single podosome and the value of F was found to be proportional to the protrusion height ( Fig. 1g,h ). Altogether, these experiments show that PFM allows precise visualization and characterization of the local protrusions that individual podosomes induce onto the substratum. 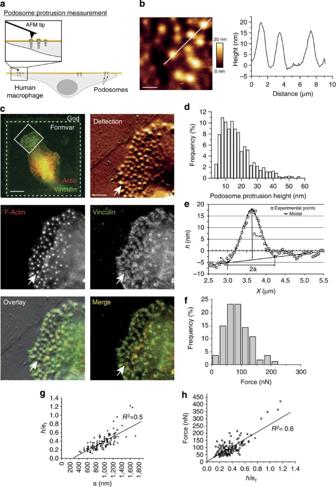Figure 1: Podosomes protrude perpendicularly to the substratum. (a) Illustration of the method for podosome protrusion measurement: PFM. At least 2 h after macrophage adhesion, AFM topographical images and height oscillation measurements of podosome protrusions were obtained on the reverse side of the Formvar sheet (for details see text;Supplementary Fig. 1;Supplementary Methods; ‘Preparation of Formvar-coated grids’; and ‘AFM experiments’ sections). (b) Representative AFM topographical image of podosome protrusions of a living human macrophage plated on a Formvar sheet. Scale bar, 2 μm. Cross-section extracted from the topographical AFM image (across the white line) depicting the heights of three podosome protrusions. (c) Correlative AFM and immunofluorescence images. The AFM deflection image (upper left panel; scale bar, 5 μm) was acquired on a living macrophage plated on Formvar sheet. The dashed line indicates the edges of the grid and a magnified view of the cell edge is shown in the upper right panel (scale bar, 20 μm). After fixation, cells were stained for F-actin and vinculin (middle and lower panels). An overlay of deflection and fluorescence microscopy is shown in the lower left panel. (d) Distribution of the height values of protrusions generated by podosomes, with a mean of 16.5±9.5 nm (n=787 podosomes from 23 cells, 12 experiments and five donors). (e) Example of the experimental profile of a podosome protrusion fitted with the model (seeSupplementary equation (4)inSupplementary Note 2) so as to determine the radiusaand the maximal heighthmaxof the protrusion. (f) Distribution of the force values generated by podosomes, with a mean of 94±59 nN,n=166 podosomes, seven experiments. (g) Linear correlation between relative protrusion heighth/efand podosome radiusa,n=144 podosomes.his the protrusion height andefthe thickness of the Formvar sheet. (h) Linear evolution of podosome protrusive forces versus relative podosome protrusion heighth/efaccording toSupplementary equation (7)inSupplementary Note 2, for the lowest values ofh/ef.n=144 protrusions, seven experiments. Figure 1: Podosomes protrude perpendicularly to the substratum. ( a ) Illustration of the method for podosome protrusion measurement: PFM. At least 2 h after macrophage adhesion, AFM topographical images and height oscillation measurements of podosome protrusions were obtained on the reverse side of the Formvar sheet (for details see text; Supplementary Fig. 1 ; Supplementary Methods ; ‘Preparation of Formvar-coated grids’; and ‘AFM experiments’ sections). ( b ) Representative AFM topographical image of podosome protrusions of a living human macrophage plated on a Formvar sheet. Scale bar, 2 μm. Cross-section extracted from the topographical AFM image (across the white line) depicting the heights of three podosome protrusions. ( c ) Correlative AFM and immunofluorescence images. The AFM deflection image (upper left panel; scale bar, 5 μm) was acquired on a living macrophage plated on Formvar sheet. The dashed line indicates the edges of the grid and a magnified view of the cell edge is shown in the upper right panel (scale bar, 20 μm). After fixation, cells were stained for F-actin and vinculin (middle and lower panels). An overlay of deflection and fluorescence microscopy is shown in the lower left panel. ( d ) Distribution of the height values of protrusions generated by podosomes, with a mean of 16.5±9.5 nm ( n =787 podosomes from 23 cells, 12 experiments and five donors). ( e ) Example of the experimental profile of a podosome protrusion fitted with the model (see Supplementary equation (4) in Supplementary Note 2 ) so as to determine the radius a and the maximal height h max of the protrusion. ( f ) Distribution of the force values generated by podosomes, with a mean of 94±59 nN, n =166 podosomes, seven experiments. ( g ) Linear correlation between relative protrusion height h/e f and podosome radius a , n =144 podosomes. h is the protrusion height and e f the thickness of the Formvar sheet. ( h ) Linear evolution of podosome protrusive forces versus relative podosome protrusion height h/e f according to Supplementary equation (7) in Supplementary Note 2 , for the lowest values of h/e f . n =144 protrusions, seven experiments. Full size image Mechanosensing activity of podosomes To explore podosome mechanosensitive properties, we first investigated how podosomes are affected by modifications of the substrate rigidity. Macrophages were plated on fibrinogen-coated glass coverslips or fibrinogen-coated polyacrylamide (PA) hydrogels of various Young’s moduli (from 0.5 to 100 kPa; Supplementary Fig. 3 ). We found, in accordance with previous reports on podosome-related structures [2] , [5] , that podosome formation was altered as the rigidity of the substratum decreased. In addition to the reduction in podosome density ( Fig. 2a ), vinculin was delocalized from the podosome ring when the Young’s modulus of the matrix was below 100 kPa and myosin IIA transverse arcs at the cell periphery were destabilized below 6.5 kPa ( Supplementary Fig. 4 ). On the basis of a methodology described previously (see ref. 8 and Supplementary Fig. 5a ), the podosome core stiffness was measured and found to be reduced from 47 to 17 kPa as the rigidity of the substratum decreased, while the podosome height remained constant with values around 550 nm ( Supplementary Fig. 5b,c ). We have previously reported that podosome stiffness oscillates periodically [8] . Here we show that podosome core softening was accompanied by smaller magnitudes and shorter time periods of stiffness oscillations ( Supplementary Fig. 5d,e ). Next we investigated the activity of myosin II on the different substrates, as this motor protein has been largely involved in mechanosensing processes [20] and previous reports have showed that it is a major regulator of podosome dynamics [8] , [18] . The level of phospho-myosin light chain (P-MLC), which corresponds to the fraction of active myosin II, was reduced on soft substrates when compared with glass ( Fig. 2b,c ). Finally, we studied the influence of substrate stiffness on the protrusion force generated by macrophages. Varying the thickness of the Formvar sheet from 30 to 80 nm increased the effective stiffness S 0 sensed by the cells from 6 to 15 nN μm −1 ( Supplementary Note 1 ). Podosome force positively correlated with increasing substrate stiffness from 29±31 to 155±84 nN ( Fig. 2d ). So, the stiffer the substrate is, the stronger the podosome protrusive forces are. Taken together, these various approaches demonstrate that, in addition to FAs, podosomes are mechanosensitive cell structures as shown by (i) modulation of the stiffness and stiffness dynamics of their cores, (ii) modulation of their density, (iii) distinct organization of their protein components, (iv) variation of myosin II activity and (v) adaptation of the protrusive forces. 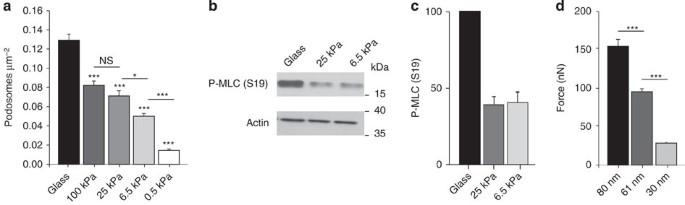Figure 2: Influence of substrate stiffness on podosome properties. (a) Quantification of podosomes on substrates of different stiffnesses. Human monocyte-derived macrophages were plated on fibrinogen-coated glass coverslip or polyacrylamide hydrogels coated with fibrinogen (Fg-PAs), then fixed and stained for F-actin (phalloidin-Alexa 488 nm). Means±s.e.m. of the number of podosomes per cell area are shown. Statistical analyses were performed by Dunnett’s multiple comparison test to compare the density of podosomes of macrophages plated on glass vs Fg-PA gels, and Tukey’s multiple comparison test to compare the density of podosomes in macrophages plated on Fg-PA gels of various stiffnesses. At least 100 cells from three different donors were measured per condition. ***P<0.001; *P<0.05; NS, nonsignificant. (b) Representative immunoblottings using antibodies directed against PhosphoSer19-MLC (P-MLC (S19)) on cell lysates from macrophages plated on glass coverslips coated with fibrinogen or on 25 kPa and 6.5 kPa Fg-PAs. (c) Means±s.e.m. of the PhosphoSer19-MLC levels normalized by actin immunoblot signal are shown. Statistical analyses were performed by Dunnett’s multiple comparison test (P<0.001). Lysates from three donors were analysed. (d) Quantification of podosome protrusive forces generated by macrophages plated on 30 nm-, 61 nm- or 80 nm-thick Formvar sheets corresponding to a stiffness of 6 nN μm−1, 12 nN μm−1and 15 nN μm−1, respectively. Means±s.e.m. of the podosome forces are shown. Statistical analyses were performed by Mann–WhitneyU-test. At least 100 protrusions from three donors were measured. ***P<0.001. Figure 2: Influence of substrate stiffness on podosome properties. ( a ) Quantification of podosomes on substrates of different stiffnesses. Human monocyte-derived macrophages were plated on fibrinogen-coated glass coverslip or polyacrylamide hydrogels coated with fibrinogen (Fg-PAs), then fixed and stained for F-actin (phalloidin-Alexa 488 nm). Means±s.e.m. of the number of podosomes per cell area are shown. Statistical analyses were performed by Dunnett’s multiple comparison test to compare the density of podosomes of macrophages plated on glass vs Fg-PA gels, and Tukey’s multiple comparison test to compare the density of podosomes in macrophages plated on Fg-PA gels of various stiffnesses. At least 100 cells from three different donors were measured per condition. *** P <0.001; * P <0.05; NS, nonsignificant. ( b ) Representative immunoblottings using antibodies directed against PhosphoSer19-MLC (P-MLC (S19)) on cell lysates from macrophages plated on glass coverslips coated with fibrinogen or on 25 kPa and 6.5 kPa Fg-PAs. ( c ) Means±s.e.m. of the PhosphoSer19-MLC levels normalized by actin immunoblot signal are shown. Statistical analyses were performed by Dunnett’s multiple comparison test ( P <0.001). Lysates from three donors were analysed. ( d ) Quantification of podosome protrusive forces generated by macrophages plated on 30 nm-, 61 nm- or 80 nm-thick Formvar sheets corresponding to a stiffness of 6 nN μm −1 , 12 nN μm −1 and 15 nN μm −1 , respectively. Means±s.e.m. of the podosome forces are shown. Statistical analyses were performed by Mann–Whitney U -test. At least 100 protrusions from three donors were measured. *** P <0.001. Full size image Molecular motors are involved in protrusion force generation We then investigated the role of myosin II-mediated contractility and actin polymerization in the regulation of protrusive force generation at podosomes. Indeed, myosin II activity has already been described to regulate the stiffness and stiffness oscillations of podosomes, as well as the tension applied to vinculin in the podosome ring [17] , [18] . The localization of myosin II in macrophage podosomes was investigated by total internal reflection fluorescence (TIRF) imaging and by immunogold labelling coupled with scanning electron microscopy (SEM) imaging. These experiments confirmed previous work [17] , [21] , [22] showing that myosin IIa is present in the F-actin cable network interconnecting podosomes ( Supplementary Fig. 6 ). To assess the role of myosin II contractility in protrusive force generation, we used two approaches: blebbistatin that directly inhibits myosin II activity and myosin II siRNAs for gene knockdown. PFM analyses showed that podosome protrusion forces were significantly reduced by 61 and 63% by blebbistatin and by myosin II silencing, respectively ( Fig. 3a–f ), with a depletion rate of myosin II of 70% ( Fig. 3c,d ). Then, to determine the role of the main myosin II-regulating kinases on force generation by podosomes, we used Y27632 and ML7 to inhibit ROCK and MLCK, respectively [23] . ML7 and Y27632 separately had modest inhibitory effects (27 and 32%, respectively) on protrusion height on Formvar. When these drugs were combined, the protrusion heights were reduced by 60% and the forces were estimated to be decreased by 69% ( Fig. 3g,h ; Supplementary Figs 7b and 8a,b ). We controlled that ML7+Y27632 treatment efficiently inhibited the phosphorylation of MLC as shown by western blots and myosin II disorganization in transverse arcs ( Supplementary Fig. 8a,c,d ). As expected, the inhibition of F-actin polymerization by cytochalasin D (CD) almost completely abolished the protrusion force of podosomes ( Fig. 3g,h ; Supplementary Fig. 7a ). Since actin polymerization is important for the generation of protrusion forces, we checked that drugs inhibiting myosin activation do not affect actin polymerization dynamics in the podosome core. To this end, fluorescence recovery after photobleaching (FRAP) experiments showed that CD treatment strongly reduced actin turnover in podosome cores, whereas it was not affected by ML7+Y27632 ( Supplementary Fig. 9a ). In a previous report, we have shown that CD and blebbistatin affected podosome height, stiffness and stiffness oscillations [8] . Here we show that the inhibition of myosin activation by Y27632+ML7 induced a slight decrease in podosome height and a 36% decrease in core stiffness and shortened oscillation period ( Supplementary Fig. 9b ) to similar levels of CD (ref. 8 ; Supplementary Fig. 9b ). Thus, myosin activity and actin polymerization are key actors of force generation by podosomes. In addition, the kinases regulating myosin II activity appear to act in concert for the regulation of force generation. 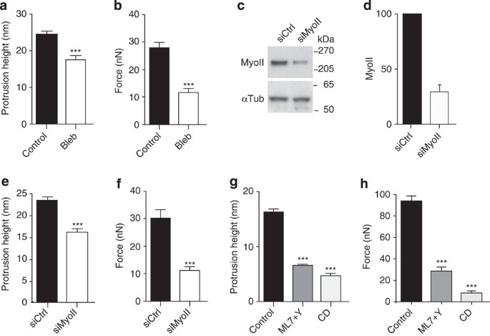Figure 3: Podosome protrusive force depends on actomyosin contractility. (a) Means±s.e.m. of podosome protrusion heights on 30 nm-thick Formvar sheets in control conditions or after blebbistatin addition are shown.t-test was used to compare protrusive heights generated by at least 200 protrusions from five donors. ***P<0.001. (b) Means±s.e.m. of podosome protrusive forces in control conditions or after blebbistatin addition are shown.t-test was used to compare protrusive forces generated by at least 100 protrusions from three donors. ***P<0.001. (c) Representative immunoblottings using antibodies directed against myosin II and αTubulin (αTub) on cell lysates from macrophages transfected with control siRNAs or siRNAs targeting myosin II. (d) Means±s.e.m. of relative myosin II levels normalized on αTubulin immunoblot signals used as a loading control are shown. Mann–WhitneyU-test (P<0.01) was used to compare relative myosin II signals in macrophages from five donors treated with indicated siRNAs. (e) Means±s.e.m. of podosome protrusion heights in control conditions or after myosin II depletion by siRNA are shown.t-test was used to compare at least 250 podosome protrusive heights generated by macrophages from five donors. ***P<0.001. (f) Means±s.e.m. of podosome protrusive forces in control conditions or after myosin II depletion by siRNA are shown. Statistical analyses were performed byt-test. 120 protrusions from three donors were measured. ***P<0.001. (g) Means±s.e.m. of protrusion heights under control conditions or after addition of ML7+Y27632 or CD are shown.t-test was used to compare at least 150 podosome protrusions in cells obtained from at least three donors. ***P<0.001. (h) Means±s.e.m. of podosome protrusive forces in control conditions or after addition of ML7+Y27632 or CD are shown.t-test and Dunnett’s multiple comparison test were used to compare at least 16 podosome protrusive forces in cells obtained from at least four donors. ***P<0.001. Figure 3: Podosome protrusive force depends on actomyosin contractility. ( a ) Means±s.e.m. of podosome protrusion heights on 30 nm-thick Formvar sheets in control conditions or after blebbistatin addition are shown. t -test was used to compare protrusive heights generated by at least 200 protrusions from five donors. *** P <0.001. ( b ) Means±s.e.m. of podosome protrusive forces in control conditions or after blebbistatin addition are shown. t -test was used to compare protrusive forces generated by at least 100 protrusions from three donors. *** P <0.001. ( c ) Representative immunoblottings using antibodies directed against myosin II and αTubulin (αTub) on cell lysates from macrophages transfected with control siRNAs or siRNAs targeting myosin II. ( d ) Means±s.e.m. of relative myosin II levels normalized on αTubulin immunoblot signals used as a loading control are shown. Mann–Whitney U -test ( P <0.01) was used to compare relative myosin II signals in macrophages from five donors treated with indicated siRNAs. ( e ) Means±s.e.m. of podosome protrusion heights in control conditions or after myosin II depletion by siRNA are shown. t -test was used to compare at least 250 podosome protrusive heights generated by macrophages from five donors. *** P <0.001. ( f ) Means±s.e.m. of podosome protrusive forces in control conditions or after myosin II depletion by siRNA are shown. Statistical analyses were performed by t -test. 120 protrusions from three donors were measured. *** P <0.001. ( g ) Means±s.e.m. of protrusion heights under control conditions or after addition of ML7+Y27632 or CD are shown. t -test was used to compare at least 150 podosome protrusions in cells obtained from at least three donors. *** P <0.001. ( h ) Means±s.e.m. of podosome protrusive forces in control conditions or after addition of ML7+Y27632 or CD are shown. t -test and Dunnett’s multiple comparison test were used to compare at least 16 podosome protrusive forces in cells obtained from at least four donors. *** P <0.001. Full size image Protrusion force oscillations at podosomes Podosomes are highly dynamic structures exhibiting periodical stiffness oscillations (ref. 8 and this report). Hence, time-lapse PFM was used to analyze the dynamics of protrusions ( Fig. 4a ; Supplementary Movies 1 and 2 ) and revealed that the protrusive force generated by a single podosome also oscillated ( Fig. 4b ). To better characterize these oscillations with a higher temporal resolution, the AFM cantilever was used as a real-time recorder by keeping the tip in contact with the top of a protrusion at a constant force of 500 pN ( Fig. 4c ). 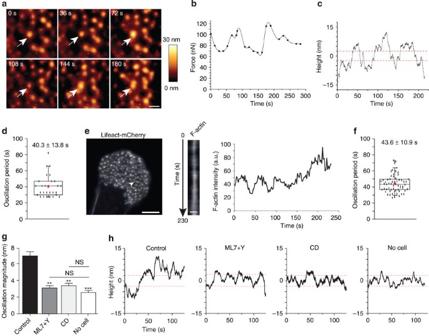Figure 4: Periodicity of podosome protrusive activity. (a) Representative time-lapse topographical AFM images of podosome protrusions, arrows point out a single protrusion whose height fluctuates over time (seeSupplementary Movie 1). Scale bar, 2 μm. (b) Representative curve of the protrusion force variations of a podosome over time in living human macrophages plated on a Formvar sheet. SeeSupplementary Note 2for details. (c) Representative curves of height fluctuations generated by podosome protrusion measured by AFM. Red lines depict the magnitude threshold (2.5 nm) defined by the ‘No cell’ mean value. See Methods, ‘AFM experiments’ section for details. (d) Quantification of podosome protrusive oscillation period measured by AFM. Fourier transform analysis was performed on 30 curves, Box-and-whisker plot and mean value (red square) are shown (mean±s.d.). Period of oscillation was not significantly different from periods of oscillation of podosome stiffness or F-actin core intensity as assessed by Tukey’s multiple comparison test on measures of the dynamics of at least 28 podosomes from three different donors. (e) (Left panel) TIRF image of a macrophage expressing Lifeact-mCherry, white arrowhead points to the podosome analysed. Scale bar, 10 μm. (Middle panel) Kymograph of Lifeact-mCherry extracted from the podosome analysed (seeSupplementary Movie 5). Scale bar, 1 μm. (Right panel) Graph depicting time-lapse oscillations of the F-actin intensity of the same podosome. (f) Quantification of podosome-core F-actin intensity oscillation period. Fourier transform analysis was performed on 44 curves such as ine, mean value (red square) is reported (mean±s.d.). (g) Means±s.e.m. of podosome protrusion oscillation magnitude in control conditions or after drug addition are shown.t-test and Dunnett’s multiple comparison test were used to compare the amplitude of podosome oscillations in cells obtained from at least four donors. ***P<0.001; **P<0.01; NS, nonsignificant. (h) Representative curves of height fluctuations generated by podosome protrusions in control macrophages and after drug treatments (ML7+Y, CD). The ‘No cell’ condition refers to height fluctuations of the Formvar sheet without cells plated on it. Red dashed lines depict the magnitude threshold defined by the ‘No cell’ mean value (threshold magnitude=2.5 nm). Figure 4: Periodicity of podosome protrusive activity. ( a ) Representative time-lapse topographical AFM images of podosome protrusions, arrows point out a single protrusion whose height fluctuates over time (see Supplementary Movie 1 ). Scale bar, 2 μm. ( b ) Representative curve of the protrusion force variations of a podosome over time in living human macrophages plated on a Formvar sheet. See Supplementary Note 2 for details. ( c ) Representative curves of height fluctuations generated by podosome protrusion measured by AFM. Red lines depict the magnitude threshold (2.5 nm) defined by the ‘No cell’ mean value. See Methods, ‘AFM experiments’ section for details. ( d ) Quantification of podosome protrusive oscillation period measured by AFM. Fourier transform analysis was performed on 30 curves, Box-and-whisker plot and mean value (red square) are shown (mean±s.d.). Period of oscillation was not significantly different from periods of oscillation of podosome stiffness or F-actin core intensity as assessed by Tukey’s multiple comparison test on measures of the dynamics of at least 28 podosomes from three different donors. ( e ) (Left panel) TIRF image of a macrophage expressing Lifeact-mCherry, white arrowhead points to the podosome analysed. Scale bar, 10 μm. (Middle panel) Kymograph of Lifeact-mCherry extracted from the podosome analysed (see Supplementary Movie 5 ). Scale bar, 1 μm. (Right panel) Graph depicting time-lapse oscillations of the F-actin intensity of the same podosome. ( f ) Quantification of podosome-core F-actin intensity oscillation period. Fourier transform analysis was performed on 44 curves such as in e , mean value (red square) is reported (mean±s.d.). ( g ) Means±s.e.m. of podosome protrusion oscillation magnitude in control conditions or after drug addition are shown. t -test and Dunnett’s multiple comparison test were used to compare the amplitude of podosome oscillations in cells obtained from at least four donors. *** P <0.001; ** P <0.01; NS, nonsignificant. ( h ) Representative curves of height fluctuations generated by podosome protrusions in control macrophages and after drug treatments (ML7+Y, CD). The ‘No cell’ condition refers to height fluctuations of the Formvar sheet without cells plated on it. Red dashed lines depict the magnitude threshold defined by the ‘No cell’ mean value (threshold magnitude=2.5 nm). Full size image We could quantify that 73% (out of 38 recordings, 13 experiments) of podosomes induced periodic oscillatory protrusions, with a time period of 40±14 s ( Fig. 4d ). Interestingly, this period was not significantly different from the period of oscillation of the podosome core stiffness (37±20 s; Fig. 4e,f ). In addition, when measuring the fluctuations of F-actin in the podosome core by TIRF time-lapse imaging of macrophage expressing Lifeact-mCherry, the amount of F-actin in the podosome core was found to oscillate with a period of 44±11 s, which was not statistically different from the period of stiffness and height oscillations ( Fig. 4e,f ; Supplementary Movie 3 ). These results strongly suggest that the force produced by a podosome oscillates in a similar manner to the stiffness and F-actin content of the podosome core. In dendritic cells, F-actin fluctuations in the podosome core have also been suggested to be controlled by actomyosin contractility [18] . We thus tested the effect on protrusion oscillations of treating macrophages with CD or with the combination of ML7 and Y27632, which had the strongest effect on protrusion force among the different strategies we used to decrease myosin activity. In macrophages, the magnitude of the oscillations of the protrusions was also reduced down to the noise background after CD or ML7+Y27632 treatment ( Fig. 4g,h ; Supplementary Movies 4 and 5 ). These results confirmed that both F-actin polymerization and myosin II activity are major actors involved in protrusion force oscillations. A model for protrusion force generation at podosomes Our results indicated that podosome mechanical activity and oscillatory behaviour are closely linked. So we designed a model to determine whether the coupling of core actin polymerization and peripheral actomyosin contraction could explain how podosomes exert periodic protrusive forces ( Supplementary Note 3 ). Our model is based on the hypothesis of force balance between the two main components: (i) a core of polymerizing actin filaments that is mainly characterized by the number of actin filaments and their stall force and the growth and retraction dynamics of this actin core that depends on the sustained stress, and (ii) a set of lateral stress fibre-like structures of actin/myosin that connect the podosome core to adhesion sites and act like active springs sustaining tensions. Note that this model only takes into account the tension produced by myosin on the lateral cables, and not the tension in these cables that might also arise from the treadmilling of actin in the podosome core, as suggested by Luxenburg et al. [24] As the value of the protrusive force generated underneath a podosome core (measured by PFM in this report) is close or larger than the maximum load of the actin filaments present in the core defined by the actin polymerization stall force, our model predicts that the coupling of the two main components can be generically unstable and tend to oscillate beyond a Hopf bifurcation ( Supplementary Note 3 ). In agreement with the effects induced by inhibition of either actin polymerization or myosin II activity, this model implies that actin filament tension generated by actomyosin contraction and actin polymerization is intimately coupled and cannot work independently to generate the podosome protrusive force. In addition, this model is in accordance with our results showing that podosome protrusive force increases with the substrate stiffness. In this study, we describe an original method named PFM designed to measure for the first time the protrusive force at single podosome sites. We report that podosomes exert a mechanosensing activity by applying a force that protrudes perpendicularly into the substratum and depends on the substrate stiffness. Applying PFM to podosomes, we measure the protrusive forces generated onto the substratum. This force depends on both F-actin polymerization and myosin II contractility. Indeed, using an actin-depolymerizing agent and several approaches to affect myosin II (drugs inhibiting myosin kinases or myosin activity directly, and siRNA-mediated myosin II depletion), all impair force generation. Interestingly, we observed that the cellular level of phospho-MLC correlates with the force intensity generated by podosomes, indicating that a significant amount of phospho-myosin is involved in that process. We also show that podosomes generate protrusions in an oscillatory manner whose period and amplitude depend on F-actin polymerization and on ROCK- and MLCK-regulated myosin II activity. The two-component model that we propose, which is based on contraction of actomyosin cables and actin core protrusion ( Fig. 5 ), is able to explain these oscillations. The oscillatory force appears to be related to the previously described periodic stiffness oscillations of the podosome core that involve the same molecular actors and display the same dynamics [8] . In addition to oscillations of podosome force and core stiffness, the actin content in podosome cores present the same periods, which likely reflects periodic actin polymerization. Oscillations of actin in the podosome core have been reported in dendritic cells and correlate with oscillations of ring proteins such as vinculin [18] . Since variations of vinculin content at adhesion complexes are known to follow traction force magnitude [25] , [26] , synchronous fluctuations of vinculin and actin in podosomes suggest that traction forces take place at the ring in a coordinated manner with protrusive force of the actin core. Thus, our data and modelling work further support the hypothesis that, at each podosome site, there is a force balance between actin polymerization at the core and actomyosin contractility at peripheral cables [7] , [17] . This is in marked contrast to FAs where only traction forces are generated and generally equilibrated cell wide [27] . When comparing the forces generated by these two cell structures on substrates with similar stiffness (12 nN μm −1 ), podosomes generate 90 nN protrusion forces and FAs generate 16 nN traction forces [25] . Although these values are of the same order of magnitude, it should be noted that distinct architectures and force generation mechanisms operate in these cell structures. An in-depth systematic comparison will be required to fully grasp the physics of these two different mechanosensing cell adhesion structures. While the main difference between the architecture of these two cell structures is the actin core protruding perpendicular to the substrate, it is interesting to question whether proteins belonging to the podosome ring such as vinculin or paxillin regulate contractility of peripheral cables in the same way as they control traction forces at FAs. 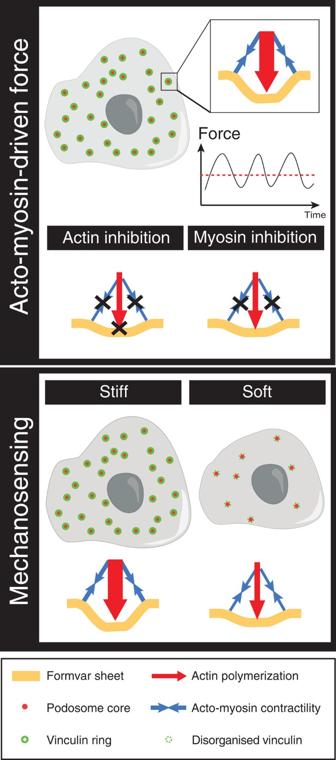Figure 5: A model for force generation at podosomes. (Upper panel) Podosomes generate periodic strains on the substratum as a result of combined pulling (blue arrows) and pushing forces (red arrows). The pulling force is mediated by the contractility of actomyosin filaments and the pushing force by actin polymerization at the plasma membrane area. On inhibition of myosin II activation or actin polymerization, podosome protrusion forces are diminished, leading to smaller strains in the substratum. (Lower panel) When macrophages adhere on soft substrates, the density of podosomes is reduced, vinculin is disorganized and podosome protrusive force is decreased. Figure 5: A model for force generation at podosomes. (Upper panel) Podosomes generate periodic strains on the substratum as a result of combined pulling (blue arrows) and pushing forces (red arrows). The pulling force is mediated by the contractility of actomyosin filaments and the pushing force by actin polymerization at the plasma membrane area. On inhibition of myosin II activation or actin polymerization, podosome protrusion forces are diminished, leading to smaller strains in the substratum. (Lower panel) When macrophages adhere on soft substrates, the density of podosomes is reduced, vinculin is disorganized and podosome protrusive force is decreased. Full size image It is noteworthy that podosomes are interconnected with neighbouring podosomes through an additional network of actin/myosin filaments, suggesting multiple scales of force equilibrium and podosome collective behaviour ( Supplementary Fig. 6 and refs 10 , 14 ). Further work is required to understand the role of these podosome networks in force generation at a whole-cell level in macrophages. Here we show that podosomes exert protrusive forces that increase with the substrate stiffness, attesting for mechanosensing properties. FAs are also mechanosensitive cell structures that exert traction forces, which increase with the substrate stiffness [25] , [28] , [29] . Thus, like FAs [30] , [31] , podosome mechanosensing activity might be important for several cell functions, including durotaxis, cell survival, response to growth factors and differentiation. In the case of macrophages, which are immune cells patrolling actively throughout the entire body, podosome protrusive force is probably an efficient way for macrophages to actively probe the viscoelastic properties of their microenvironment and proceed to optimal migration modes [9] . The conceptual and technical novelty of PFM will pave the way for the study of protrusive force-mediated mechanosensing in macrophages, but also in other protrusion-dependent processes such as cancer cell invasion [32] , antigen recognition [33] , frustrated phagocytosis [34] and diapedesis [35] . Cell culture and treatment with drugs and siRNA Monocytes from healthy donors were isolated by centrifugation through Ficoll–Hypaque, resuspended in ice-cold buffer composed of phosphate-buffered saline (PBS), 2 mM EDTA and 0.5% fetal calf serum (FCS) at pH 7.4 and magnetically sorted by CD14 magnetic microbeads (Miltenyi Biotec, Auburn, CA). Monocytes were then distributed on glass coverslips at 2 × 10 6 in six-well plates in RPMI 1640 containing 10% heat-inactivated FCS, antibiotics and 20 ng ml −1 macrophage colony-stimulating factor (PeproTech, Rock Hill, NJ) and incubated at 37 °C in humidified 5% CO 2 atmosphere. The culture medium was renewed on the third day. After 7 days of differentiation, human monocyte-derived macrophages (hMDMs) were trypsinized (Invitrogen) and seeded at 4.5 × 10 4 cells cm −2 on glass coverslips, hydrogels and on Formvar-coated grids in RPMI medium containing antibiotics. For western blot experiments, cells were seeded at 1 × 10 6 cells per well in six-well plates. For immunofluorescence imaging and AFM experiments, macrophages were plated for 1 h on glass coverslips or PA hydrogels in RPMI medium without FCS supplemented with antibiotics, and then in complete medium. Cells were observed 20 min after addition of 50 μM blebbistatin (Sigma), a concentration which fully inhibits myosin II [36] , [37] . ML7 (Calbiochem) and Y27632 (VWR International) or CD (Sigma) were added to the medium 3 h after plating the cells, at 10 and 20 μM or 2 μM, respectively. Dimethylsulphoxide was used as a control for blebbistatin, ML7+Y27632 and CD. Cells for immunofluorescence experiments were analysed by AFM from 15 min to 1 h after addition of blebbistatin, ML7+Y27632 or CD and then fixed. Correlative AFM topographical image and immunostaining show that the chosen drug concentration (ML7+Y27632) impacts the global cell morphology but does not abolish the presence of podosomes (ML7+Y27632; Supplementary Fig. 8 , CD as described in ref. 8 ). hMDMs were transfected at day 7 of differentiation with 166 nM of a control siRNA or myosin IIA (83 nM)+myosin IIB (83 nM) siRNAs (Dharmacon, Illkirch) using the Hiperfect system (Qiagen) [38] . The mix of Hiperfect and siRNA was incubated for 15 min at room temperature and then added drop by drop to the cells. The following siRNAs were used: ON-TARGET plus SMART pool siRNA, MYH9 sequences: 5′-GUAUCAAUGUGACCGAUUU-3′; 5′-CAAAGGAGCCCUGGCGUUA-3′; 5′-GGAGGAACGCCGAGCAGUA-3′; 5′-CGAAGCGGGUGAAAGCAAA-3′. ON-TARGET plus SMART pool siRNA, MYH10 sequences: 5′-GGAAGAAGCUCGACGCGCA-3′; 5′-GAGCAGCCGCCAACAAAUU-3′; 5′-GGGCAACUCUACAAAGAAU-3′; 5′-CCAAUUUACUCUGAGAAUA-3′. Cells were observed 10 days after transfection. Preparation of Formvar-coated grids The film casting device (Electron Microscopy Science, EMS #71305-01) was used for casting support films onto electron microscope grids. Two hundred mesh nickel grids (EMS) were used. To ensure good film adhesion, the grids were first washed two times and sonicated in acetone, then placed onto a lint-free filter paper and allowed to dry. Glass microscope slides were cleaned with fibre-free tissues and ethanol. Clean slides were dipped into a Formvar solution of 0.5% (w/v) ethylene dichloride (EMS) for a few seconds and the Formvar solution was emptied from the film casting device using a calibrated downwards flow. Different thicknesses of Formvar sheets are obtained on the glass slides using distinct flow rates for the drainage of the Formvar solution. The slides were dried in a vertical position and the film was detached from the slide by contact with water and was left floating at the surface. Grids were arranged on floating films, picked up coated with the film onto another glass slide and then air dried. AFM experiments A NanoWizard II or a NanoWizard III AFM (JPK Instruments) mounted on an inverted optical microscope (Axiovert 200, Carl Zeiss) were used for both cell imaging and force spectroscopy. Silicon nitride cantilevers (MLCT-AUHW, Veeco Instruments) with a nominal spring constant of 0.010 N m −1 were used in all experiments, except when indicated for the quantification of the mechanical properties of the Formvar sheet in Supplementary Note 1 . For each cantilever, the spring constant was determined using the thermal noise method [39] . To ensure reproducibility in force application, the cantilever sensitivity and spring constant were calibrated before each experiment using the JPK Instrument software. The optical microscope was used to select the desired cell and to position the AFM tip. All AFM images and measurements were obtained in contact mode in liquid. AFM Imaging and height measurements . For AFM analysis of living cells seeded on glass coverslips, on PA gels coated with fibrinogen or on Formvar-coated grids, a temperature-controlled sample holder was used (BioCell, JPK Instruments) and the culture medium (RPMI 1640 containing 10% FCS and antibiotics) was supplemented with 10 mM HEPES. pH 7.4 (Sigma). Living cells were imaged with a pixel resolution of 256 or 512 pixels at line rate around 2–3 Hz. For AFM topographical characterization of the Formvar-coated grids, images were recorded with a pixel resolution from 32 to 256 pixels at line rate from 10 to 30 Hz depending on the scanned area. The imaging parameters were carefully monitored to achieve a good contrast with scanning forces typically lower than 1 nN. AFM images were analysed using the JPK Image Processing software. For height measurements of podosomes, a linear plane fit on the topographical image was performed to remove the tilt angle due to the sample mounting, and the surface of the glass coverslip or PA gel was taken as the zero reference of the sample height. For height measurements of podosome-induced protrusions, a polynomial correction by line and surface (order 3) of the topographical image was performed to level the image. Values extracted from the corrected topographical images were then treated using Origin software (OriginLab). For thickness measurements of the Formvar sheet, after removing Formvar-coated grids, the Formvar sheet remaining on the glass slide was imaged in contact mode by AFM. Thicknesses of the Formvar sheets were measured taking the glass coverslip surface as the height reference ( Supplementary Fig. 1b ). Except when mentioned, Formvar sheets used in most experiments were 61 nm thick. Intermittent time-resolved stiffness measurements . Stiffness measurements were derived from force-versus-distance profiles (extend curves) using the dedicated JPK software. Briefly, at different selected points of the cell, the deflection of the cantilever is recorded when the AFM tip is approaching and converted into force using a pre-calibration curve obtained on a hard substrate. After tip contact with the cell surface, the indentation of the cell induces a constant increase in the force sensed by the cantilever. When the force reaches a value of 500 pN, the tip is automatically retracted and a new force–distance curve can be recorded at the same site or at a new location. The determination of elastic modulus E from the force–distance curves was then performed using a modified Hertz model [8] , [40] , [41] . A first AFM image was recorded from the sample and the topographical image was used to select the points for stiffness measurements. Then, a series of 120 curves was performed for each point at 2 Hz (1 s per approach/retract event), and the Young’s modulus was calculated for each extended curve. Each data series whose residual error on the fitting of force curves with the Hertz model was above 10 pN was discarded [8] . After stiffness measurements, the podosome state was estimated by AFM imaging and experiments in which the podosomes that had disappeared were discarded. Mean values of Young’s modulus of podosomes in living human macrophages were extracted from time-lapse stiffness measurements. The validity of podosome stiffness measurement on macrophages plated on PA hydrogels was carefully examined by verifying that the measured value did not depend on the selected AFM tip indentation depth, as previously reported [8] . Briefly, we observed that, independently of the gel stiffness, a plateau in the measured E value was reached beyond a similar indentation depth, that is, around 80 nm. Moreover, this threshold value of 80 nm was identical when macrophages were plated on glass. This minimal indentation depth probably corresponds to the thickness of the cell components overlying the top of the podosome core. As this threshold of 80 nm did not depend on the rigidity of the substrate, we could confirm that the differences of measured Young’s modulus are representative of real podosome stiffness variations and are not due to substrate artefacts ( Supplementary Fig. 4b ). Real-time recording of the height of the podosome-induced protrusions . First, the Formvar-coated grid plated with macrophages was placed over a glass coverslip and maintained between two strips of doubled-sided adhesive tape ( Supplementary Fig. 1a ). The device was then introduced in the temperature-controlled sample holder (37 °C, BioCell, JPK Instruments) and the culture medium (RPMI 1640 containing 10% FCS and antibiotics) was supplemented with 10 mM HEPES, pH 7.4 (Sigma). The AFM cantilever was calibrated on the glass coverslip as described in ‘Intermittent time-resolved stiffness measurements’ in order to be able to transform the photodiode signal into an applied force. First, an AFM image of the Formvar sheet was recorded to set the measurement point at the location of the podosome-induced protrusion. The AFM tip was then held in contact with the Formvar sheet at constant force (500 pN) and the tip deflection was recorded during at least 120 s. The raw curve obtained was then linearized to account for the thermal drift of the cantilever during the recording time. Protrusion period was then estimated using Fourier transform analysis (OriginLab). The oscillation magnitude of podosome-induced protrusions refers in this paper to the s.d. value of the linearized curve. Fabrication of fibrinogen-coated PA hydrogels PA hydrogel preparation on aminosilanized glass coverslips was adapted from ref. 42 . Briefly, glass coverslips were treated using 3-aminopropyl trimethoxysilane (Sigma) and covered with various solutions containing a ratio of acrylamide and bis-acrylamide (Sigma) to tune the elastic modulus as desired (see Supplementary Table 1 ) and 0.15% TEMED and 1% ammonium persulfate in distilled water to allow reticulation. Before their complete reticulation, hydrogels were covered with a glass coverslip. Once full polymerization was completed, top coverslips were discarded and hydrogels were washed with 50 mM HEPES buffer at pH 8.4. Fibrinogen (human plasma, Sigma) was covalently linked at the surface of the PA gels using the photoactivable heterobifunctional reagent sulfosuccinimidyl-6-(4'-azido-2'-nitrophenylamino) hexanoate (sulfo-SANPAH, VWR). After photoactivation with ultraviolet light, a 0.1 mg ml −1 fibrinogen solution (in 50 mM HEPES buffer) was incubated onto the PA hydrogels overnight at 4 °C. Before use, PA hydrogels were washed three times with HEPES buffer (50 mM, pH 8.4), incubated for 30 min at 37 °C in cell culture medium before plating cells. Rheology of PA hydrogels Gel response to oscillatory shear was measured using a rheometer (Advanced Rheometer AR1000) equipped with a cone (diameter: 40 mm; angle: 2°)/flat-plate geometry. The plate was first refrigerated at 10 °C. PA solution (600 ml) was prepared as above at 4 °C, then placed in the centre of the lower plate. The plate was heated to 37 °C, and the sample was left undisturbed for 5 min to allow reticulation. Then, PA hydrogels were subjected to oscillatory shear by rotating the cone around its axis with a maximum strain of 0.25. Both the shear storage modulus ( G′ ) and the shear loss modulus ( G′′ ) were measured in the linear viscoelastic domain as a function of the frequency of the angular velocity from 0.1 to 10 Hz (see Supplementary Fig. 3 ). Assuming that the shear loss modulus values were negligible compared with G′ values (inferior to 1.5% of the G′ value), the shear modulus G (| G|*=(G′ 2 +G′′ 2 ) 1/2 ) could be taken as G = G′ . Elastic ( E ) and shear moduli ( G ) are related by the following relation: E =2 G (1+ ν ), where ν is the Poisson ratio (assumed to be 0.5 for PA [43] ). As a consequence, PA elastic modulus could be calculated as three times its shear modulus [44] . Fibrinogen coating on glass Coverslip coating with 0.1 mg ml −1 human fibrinogen (Sigma-Aldrich) was adapted from ref. 45 . In brief, glass coverslips were coated with 50 μg ml −1 poly- L -lysine (Sigma-Aldrich) for 20 min, washed with PBS and fixed with 0.5% glutaraldehyde (EMS) for 15 min. After three washes, the coverslips were incubated for 10 min with the fibrinogen solution in PBS. After washing with PBS, coverslips were incubated in 5 mg ml −1 sodium borohydride for 3 min, washed three times in PBS and finally incubated in 2 ml of culture medium before adding the cells. Western blot analysis Cells were washed 4 h after plating (for all tested conditions) in PBS containing a 2 mM orthovanadate solution. Then, cell lysates were obtained by adding 100 μl of boiling 2 × Laemmli buffer containing phosphatase inhibitors (2 mM orthovanadate, 5 mM NaF) on cell monolayers. Samples were boiled for 5 min. For phospho-MLC analysis, cell proteins (20 μg) were subjected to electrophoresis in 15% SDS–PAGE gels, and transferred onto a nitrocellulose membrane. For myosin II analysis, cell proteins were subjected to electrophoresis in NuPAGE Novex 3–8% Tris-Acetate, and transferred onto a polyvinylidene difluoride membrane (GE Healthcare). Then, membranes were saturated with 3% bovine serum albumin in Tris-buffered saline for 1 h, and incubated with anti-tubulin (Sigma, 1/10,000), anti-actin (1/40,000), anti-MLC, anti-(p-Ser19)-MLC antibodies (1/500; Cell Signaling Technology) or anti-myosin IIA (Covance, 1/500) overnight at 4 °C. Then, primary antibodies were revealed using an horseradish peroxidase-coupled anti-mouse (Sigma) or anti-rabbit (Cell Signaling Technology, 1/10,000) secondary antibody for 1 h. Finally, horseradish peroxidase activity was revealed using a chemiluminescence kit (Amersham) according to the manufacturer’s instructions. For quantification, blots were normalized by the expression of actin or tubulin used as a loading control. Fluorescence imaging For immunofluorescence, cells were fixed for 1 h at room temperature in 3.7% (w/v) paraformaldehyde solution containing 15 mM sucrose and permeabilized with 0.1% Triton X-100 (Sigma). F-actin was visualized with AlexaFluo 488-, AlexaFluo Texas red- or AlexaFluo 355-phalloidin (Invitrogen, 1/500), vinculin was revealed with a monoclonal anti-vinculin antibody (Sigma, 1/500) and myosin IIA was stained with polyclonal anti-MHC-A (Covance, 1/500). Wide-field fluorescence images were acquired with a Leica DMRB microscope equipped with × 40/1.0 or × 100/1.4 oil immersion objectives and a Cool-SnapHQ camera (Roper Scientific) driven by MetaVue software (Roper Scientifics). Confocal and TIRF images were acquired using the × 60/1.4 and × 60/1.49, respectively, with an Olympus FV1000 microscope. For analysis of F-actin oscillations shown in Fig. 4e , cells were transfected with Lifeact-mCherry and Paxillin-EGFP using a Neon MP 5000 electroporation system (Invitrogen) with the following parameters: two 1,000 V, 40 ms pulses, with 1 μg of DNA for 2 × 10 5 cells. Cells were plated in eight-well Lab-Tek Chamber Slide System (Thermo Scientific) and imaged by TIRF microscopy every 2 s during over 5 min within 24 h of transfection. The dynamics of podosomes was analysed with Fiji software. Briefly, the F-actin image was segmented using the ‘auto local threshold' function of the software to detect podosome cores at each time. Around each of these podosomes, a 4-μm 2 -large region centred on the core was duplicated into a stack, and then registered with the MultiStackReg plugin. Each podosome was thus followed individually until more than one podosome was detected inside this region. Only F-actin cores that were correctly segmented during at least 200 s were considered for analysis. The F-actin content of podosomes was obtained by multiplying the F-actin segmented area by the mean fluorescent intensity without the mean fluorescent background. Fast Fourier Transform analysis of F-actin content fluctuations along time was performed with Excel software. For FRAP analysis, human primary macrophages were transfected with mRFP-actin (kindly provided by S. Linder) and plated in a glass-based chamber (Lab-Tek) 24 h before the experiment. FRAP was performed on a LSM710 confocal microscope (Zeiss) using a dedicated FRAP module included in the ZEN software. The microscope was equipped with a × 40 1.3 oil objective and a 37 °C and 5% CO 2 incubator. The 561 nm laser line was used for both imaging and bleaching. Images were acquired every 5 s with a pixel dwell of 9 μs. Podosomes were delimited by creating circular regions of 1.05 μm diameter and bleached sequentially to obtain a 50±10% decrease in fluorescence. Recovery and control curves (fluorescence intensity extracted from a non-bleached region) were measured with ImageJ and exported and fitted following Soumpasis equation [46] in Excel. t 1/2 values were calculated from the fit. Scanning electron microscopy For SEM observations of podosomes, macrophages were incubated in distilled water containing 10 μg ml −1 phalloidin (Sigma) at 37 °C for 40 s, and unroofed by flushing during 10 s before being fixed for 1 h in a 2.5% glutaraldehyde in 0.1 M cacodylate buffer (pH 7.4, EMS). For localization of myosin IIA at podosomes, unroofed cells were sequentially incubated with polyclonal anti-MHC-A (Covance, 1/100) and goat anti-rabbit coupled to 10 nm gold beads (Aurion). Preparations were then washed three times for 5 min in 0.2 M cacodylate buffer (pH 7.4), post-fixed for 1 h in 1% (wt/vol) osmium tetroxide in 0.2 M cacodylate buffer (pH 7.4) and washed with distilled water. Samples were dehydrated through a graded series (25–100%) of ethanol, transferred in acetone and subjected to critical point drying with CO 2 in a Leica EMCPD300. Dried specimens were sputter coated with 3 nm platinum (in Supplementary Fig. 6a ) or chromium (in Supplementary Fig. 6c ) with a Leica EM MED020 evaporator and were examined and photographed with a FEI Quanta FEG250. How to cite this article: Labernadie, A. et al. Protrusion force microscopy reveals oscillatory force generation and mechanosensing activity of human macrophage podosomes. Nat. Commun. 5:5343 doi: 10.1038/ncomms6343 (2014).